Pronounced interannual variability in tropical South Pacific temperatures during Heinrich Stadial 1 The early last glacial termination was characterized by intense North Atlantic cooling and weak overturning circulation. This interval between ~18,000 and 14,600 years ago, known as Heinrich Stadial 1, was accompanied by a disruption of global climate and has been suggested as a key factor for the termination. However, the response of interannual climate variability in the tropical Pacific (El Niño-Southern Oscillation) to Heinrich Stadial 1 is poorly understood. Here we use Sr/Ca in a fossil Tahiti coral to reconstruct tropical South Pacific sea surface temperature around 15,000 years ago at monthly resolution. Unlike today, interannual South Pacific sea surface temperature variability at typical El Niño-Southern Oscillation periods was pronounced at Tahiti. Our results indicate that the El Niño-Southern Oscillation was active during Heinrich Stadial 1, consistent with climate model simulations of enhanced El Niño-Southern Oscillation variability at that time. Furthermore, a greater El Niño-Southern Oscillation influence in the South Pacific during Heinrich Stadial 1 is suggested, resulting from a southward expansion or shift of El Niño-Southern Oscillation sea surface temperature anomalies. Near the onset of the last glacial termination, a massive discharge of icebergs marked the cold Heinrich Stadial 1 (HS1) interval in the North Atlantic region that was accompanied by a weaker Atlantic meridional overturning circulation (AMOC) [1] , [2] , [3] . The extreme climate conditions during this interval were communicated throughout the Northern Hemisphere into the tropics through changes in ocean and atmospheric circulation, resulting in a weakening of the Asian Monsoon and a southward shift of the Intertropical convergence zone [3] . These changes were accompanied by a southward shift of the Southern Hemisphere westerlies, which has been suggested as crucial in driving the rise of atmospheric CO 2 during the last termination [3] , [4] . The impact of HS1 on interannual climate variability in the tropical Pacific, however, is poorly known, largely because of the low temporal resolution of available proxy records. However, a better knowledge of the glacial dynamics of the dominant mode of Pacific atmosphere-ocean variability on interannual timescales, the El Niño-Southern Oscillation (ENSO), is critical regarding its dramatic global climate and socioeconomic impacts and difficult to predict behaviour under future climate change [5] , [6] . Moreover, HS1 provides an opportunity to validate climate models under extreme boundary conditions of the past, which can help to constrain more reliable projections of future ENSO variability [5] , [6] . Reconstructions from tropical Pacific sediments indicate an ambiguous pattern of ENSO dynamics with respect to HS1 (refs 7 , 8 ). This may reflect difficulties associated with the interpretation of ENSO variability from records that do not resolve interannual variability, or different aspects or timescales of ENSO captured by the individual reconstructions. In contrast, seasonally resolved records from fossil shallow-water corals were successfully used to reconstruct interannual ENSO variability in the tropical Pacific during the last glacial [9] , but represent short intervals older than 38,000 years only. A few coral records are available for intervals of the last glacial termination [10] , [11] , [12] , [13] , [14] , but are too short to document significant interannual ENSO variability. In modern observations, ENSO variability is described by monitoring tropical Pacific sea surface temperature (SST) [15] . However, proxy records of interannual tropical Pacific SST variability during HS1 do not exist, largely because fossil reefs of that age are difficult to access as global sea level stood some 100 m lower than today [16] . Here we present results from a fossil coral recovered by Integrated Ocean Drilling Program (IODP) Expedition 310 in the central tropical South Pacific 113 m below present sea level [17] . In the skeleton of this coral, we analyse the Sr/Ca temperature proxy at monthly resolution representing an interval of more than 2 decades during HS1. We show that significant interannual SST variability at typical ENSO periods occurred at Tahiti, which is different from today. Our results suggest a greater ENSO influence in the South Pacific at that time, and indicate that ENSO was operating and that interannual ENSO variability was pronounced during HS1. Our results are consistent with climate model simulations that indicate enhanced ENSO variability during this interval of the last glacial termination, which was characterized by extreme cold conditions in the North Atlantic and a weakening of the AMOC. Coral preservation and age Fossil Porites coral (310-M0024A-11R-2W 1-62) was recovered from 21 m below sea floor at the outer fore-reef slope off Tiarei on the north side of Tahiti island (French Polynesia, IODP Hole M0024A, 149° 24.2358′ W, 17° 29.2918′ S; Fig.1 ) [17] . X-radiography of the slabbed coral core reveals skeletal density banding and a continuous upward growth at a rate of ~2.0 cm per year, consistent with the 60-cm-high colony being drilled in growth position. Powder X-ray diffraction, petrographic thin sections, scanning electron microscopy (SEM) and micron-scale laser ablation (LA)-ICP-MS analyses indicate that the aragonitic coral skeleton is well preserved ( Supplementary Methods and Supplementary Figs S1–S7 ). Two highly consistent U-Th ages indicate that the coral grew 14.994±0.025 thousand years before the present (kyr BP; 'present' is defined as AD 1950) [18] (see Methods and Supplementary Table S1), a few centuries before the onset of the Bølling warming at 14.642 kyr BP (maximum counting error 0.186 kyr) [19] that followed the cold HS1 in the North Atlantic ( Fig. 2 ). Three modern Tahiti Porites corals were used as a benchmark with respect to seasonality and mean conditions. Our modern coral (TAH-95) drilled in June 1995 at 4–5 m water depth on the fore-reef slope of the Papeete barrier reef (Faré Uté) on the north side of Tahiti provides a short record for proxy calibration with local SST (see Methods and Supplementary Fig. S8 ). The two longer records of modern corals from the Teahupoo (TH1) and Vairao (TH2) lagoons in southeastern Tahiti [20] were used as a benchmark with respect to interannual variability. 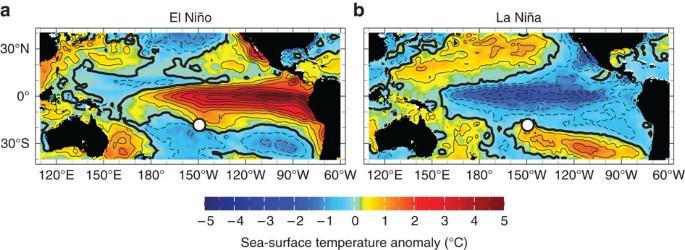Figure 1: Maps of the Pacific Ocean. Composite maps of sea-surface temperature anomalies35for moderate to strong (a) El Niño and (b) La Niña events during the period 1982–2008 (November–February). The location of Tahiti (and Integrated Ocean Drilling Program site M0024) in the tropical South Pacific is indicated by the white dot. Figure 1: Maps of the Pacific Ocean. Composite maps of sea-surface temperature anomalies [35] for moderate to strong ( a ) El Niño and ( b ) La Niña events during the period 1982–2008 (November–February). The location of Tahiti (and Integrated Ocean Drilling Program site M0024) in the tropical South Pacific is indicated by the white dot. 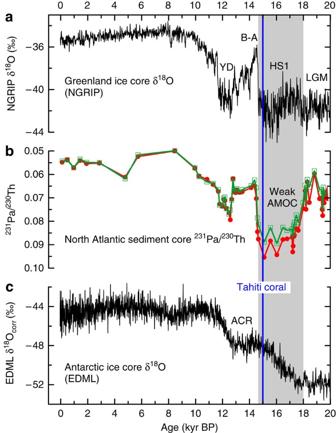Figure 2: Tahiti coral age and North Atlantic and Antarctic climate reconstructions. (a) Greenland ice core δ18O (North Greenland Ice Core Project, NGRIP), an air temperature proxy58(GICC05 age scale19relative to AD 1950). Younger Dryas (YD), Bølling-Allerød (B-A), Heinrich Stadial 1 (HS1, grey bar) (as defined in refs3,59) and late Last Glacial Maximum (LGM) are indicated. (b) North Atlantic sediment core231Pa/230Th, an AMOC strength proxy2. (c) Antarctic ice core δ18O (EPICA Dronning Maud Land, EDML), an air temperature proxy21. Antarctic Cold Reversal (ACR) is indicated. The blue bar indicates the U-series age of the fossil Tahiti coral. For clarity, bar width represents twice the dating uncertainty. All ages are given in thousand years before present (kyr BP), where 'present' refers to AD 1950. Full size image Figure 2: Tahiti coral age and North Atlantic and Antarctic climate reconstructions. ( a ) Greenland ice core δ 18 O (North Greenland Ice Core Project, NGRIP), an air temperature proxy [58] (GICC05 age scale [19] relative to AD 1950). Younger Dryas (YD), Bølling-Allerød (B-A), Heinrich Stadial 1 (HS1, grey bar) (as defined in refs 3 , 59 ) and late Last Glacial Maximum (LGM) are indicated. ( b ) North Atlantic sediment core 231 Pa/ 230 Th, an AMOC strength proxy [2] . ( c ) Antarctic ice core δ 18 O (EPICA Dronning Maud Land, EDML), an air temperature proxy [21] . Antarctic Cold Reversal (ACR) is indicated. The blue bar indicates the U-series age of the fossil Tahiti coral. For clarity, bar width represents twice the dating uncertainty. All ages are given in thousand years before present (kyr BP), where 'present' refers to AD 1950. Full size image Coral Sr/Ca record Our 15.0 kyr BP Tahiti coral provides an ultrahigh-resolution snapshot of tropical Pacific climate variability during HS1. In the western tropical Pacific and Antarctica, this interval was characterized by deglacial warming [21] , [22] , whereas the conditions that prevailed in the eastern tropical Pacific are still debated [23] , [24] ( Fig. 2 and Supplementary Fig. S9 ). The Sr/Ca ratios in coral skeletons are an established proxy for SST variability [10] , [11] , [25] , [26] , [27] , [28] . Here we present a monthly resolved Sr/Ca-based SST reconstruction for a time window of 22 years generated from our HS1 coral ( Fig. 3a ), which is exceptionally long given the corals' age and recovery method. The reconstruction shows clear annual cycles indicating SST seasonality with an amplitude that is not different from today ( Fig. 3a ; Supplementary Fig. S10 ). Furthermore, a lowering of mean SST relative to today is suggested ( Supplementary Fig. S9 ). The most striking result, however, is that spectral analysis reveals significant variance in the SST reconstruction at interannual periods of 2 and 5 years ( Fig. 3a ). This finding indicates that pronounced interannual variability at typical ENSO periods occurred in tropical South Pacific SST at 15.0 kyr BP. Our result strongly suggests that ENSO was active during HS1, and had an influence on interannual SST variability around Tahiti. Interestingly, the ENSO influence on Tahiti SST is weak and non-stationary at present. This results from the fact that, today, Tahiti is located near the nodal line of ENSO-induced SST anomalies in the Pacific, resulting in anomalies close to zero and of varying sign during both El Niño and La Niña events ( Fig. 1 ). Consequently, modern Tahiti coral Sr/Ca-based SST records [20] do not reveal significant variance at typical ENSO periods ( Fig. 3b ), in contrast to our HS1 coral Sr/Ca record. 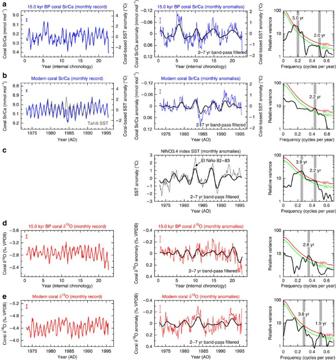Figure 3: Monthly Sr/Ca and δ18O records of TahitiPoritescorals. Monthly coral Sr/Ca records (left panel), 2–7 year Gaussian band-pass filtering of monthly anomaly records (middle panel) and multitaper method spectral analysis (significance relative to a red noise null hypothesis determined with the robust method of noise background estimation60; number of tapers, 3; bandwidth parameter, 2; 95 and 99% confidence levels indicated; significant spectral peaks labelled) of detrended and normalized monthly anomaly records (right panel) for (a) a Heinrich Stadial 1 coral (15.0 kyr BP) and (b) a modern coral20(average record of cores TH1 and TH2 drilled from two individual colonies). Local Tahiti SST is available from 1979–1991 (ref.31). There is a limitation of coral Sr/Ca in recording the very high SST of 1984. Coral-based SST anomalies (respective mean was subtracted), using our seasonal Tahiti coral Sr/Ca-SST relationship of 0.057 mmol mol−1per 1 °C are shown. (c) Monthly NINO3.4 index35(SST anomalies in the central equatorial Pacific: 170°–120°W, 5°N–5°S) and corresponding band-pass filtering and spectral analysis. (d,e) As in (a,b), but for monthly coral δ18O records. The age of the fossil coral is given in thousand years before present (kyr BP), where 'present' refers to AD 1950. Figure 3: Monthly Sr/Ca and δ 18 O records of Tahiti Porites corals. Monthly coral Sr/Ca records (left panel), 2–7 year Gaussian band-pass filtering of monthly anomaly records (middle panel) and multitaper method spectral analysis (significance relative to a red noise null hypothesis determined with the robust method of noise background estimation [60] ; number of tapers, 3; bandwidth parameter, 2; 95 and 99% confidence levels indicated; significant spectral peaks labelled) of detrended and normalized monthly anomaly records (right panel) for ( a ) a Heinrich Stadial 1 coral (15.0 kyr BP) and ( b ) a modern coral [20] (average record of cores TH1 and TH2 drilled from two individual colonies). Local Tahiti SST is available from 1979–1991 (ref. 31 ). There is a limitation of coral Sr/Ca in recording the very high SST of 1984. Coral-based SST anomalies (respective mean was subtracted), using our seasonal Tahiti coral Sr/Ca-SST relationship of 0.057 mmol mol −1 per 1 °C are shown. ( c ) Monthly NINO3.4 index [35] (SST anomalies in the central equatorial Pacific: 170°–120°W, 5°N–5°S) and corresponding band-pass filtering and spectral analysis. ( d , e ) As in ( a , b ), but for monthly coral δ 18 O records. The age of the fossil coral is given in thousand years before present (kyr BP), where 'present' refers to AD 1950. Full size image Coral δ 18 O record The HS1 coral δ 18 O record reveals only weak variance at ENSO periods ( Fig. 3d ). This is not necessarily in conflict with the Sr/Ca results as δ 18 O reflects variations in both temperature and δ 18 O seawater , which is closely related to salinity. Modern coral δ 18 O records from the Tahiti region reveal significant variance at ENSO periods of 2–5 years, although the ENSO signal is not well pronounced [20] , [29] ( Fig. 3e ). This δ 18 O ENSO signal results from the northeastward (southwestward) shift of the South Pacific Convergence Zone (SPCZ) of enhanced precipitation and the westward (eastward) movement of the southwestern tropical Pacific salinity front during El Niño (La Niña) events [30] . The HS1 coral lived in a water depth of ≤10 m, more likely in ≤5 m (ref. 18 ), similar to our modern Tahiti corals. Consequently, less variance at ENSO periods relative to today in the HS1 coral δ 18 O record can be interpreted as a change in the influence of the SPCZ and/or the salinity front on Tahiti δ 18 O seawater during HS1. Sr/Ca records of three modern Tahiti Porites corals indicate an annual SST cycle varying from 2.2 to 3.2 °C, satisfactorily documenting the observed annual cycle of 2.6 °C (ref. 31 ). This is consistent with results from other locations, showing that the seasonal amplitude between colonies is reproducible [27] . We therefore consider our result of an annual SST cycle of 2.7 °C at 15.0 kyr BP, which is similar to today, as robust ( Supplementary Fig. S10 ). Our estimates of a reduction in mean SST by 3.5 °C relative to today, using our seasonal Tahiti coral Sr/Ca-SST relationship or by only 2.4 °C, using a possibly more suitable relationship for mean Indo-Pacific SST changes [32] , however, have relatively large uncertainties. As commonly observed at various locations [27] , [28] , [33] , between-colony offsets in mean Sr/Ca are evident among the modern Tahiti corals ( Supplementary Methods and Supplementary Fig. S9 ). Taking into account the error induced by these offsets [33] results in estimates of 3.5±2.8 °C or 2.4±2.0 °C for the cooling at 15.0 kyr BP, depending on the applied coral Sr/Ca-SST relationship. Furthermore, correcting for potential changes in seawater Sr/Ca on glacial–interglacial timescales [34] leads to smaller cooling estimates, partly in agreement with foraminiferal Mg/Ca and alkenone SST reconstructions from the equatorial Pacific [22] , [23] , [24] , but adds additional uncertainties. Clearly, Sr/Ca records from more than one coral would be necessary [33] to robustly estimate mean Tahiti SST at 15.0 kyr BP. It is important to note that our major result, the stronger than modern ENSO signal in Tahiti SST during HS1 ( Fig. 3a,b ), does not necessarily mean that the interannual variability of the entire ENSO phenomenon was stronger at that time, as the difference can be explained by a shift in the nodal line of ENSO-induced SST anomalies relative to Tahiti ( Fig. 1 ). Our results imply Tahiti was located permanently either in the region of positive or of negative SST anomalies during El Niño events, in the time window represented by the HS1 coral. We surmise that a southwestward shift of the nodal line rather than a northeastward shift is more likely, which would have placed Tahiti in the region of positive SST anomalies during El Niño events. This claim is based on four high-amplitude interannual warm events (anomalies ≥1 °C) in the HS1 SST reconstruction ( Fig. 3a ), with the most prominent event (~1.5 °C) of two years duration being supported by the U/Ca SST proxy ( Supplementary Methods and Supplementary Fig. S11 ). Such high SST amplitudes are characteristic for modern El Niño events in the equatorial Pacific ( Fig. 3c ), whereas the influence and amplitude of ENSO in the subtropical southwestern Pacific is much weaker ( Fig. 1 ). Moreover, the standard deviation of reconstructed Tahiti monthly SST anomalies in the 2–7 year ENSO band for HS1 is 28% higher than the modern case, which is similar to that observed ~10° further north today [35] . However, we note that our reconstructed difference in ENSO variability is not inconsistent with long-term changes in ENSO behaviour observed in unforced climate model simulations [36] . Nevertheless, our results indicate a greater influence of interannual ENSO variability on tropical South Pacific SST during HS1, and suggest a southward expansion or shift of ENSO SST anomalies at that time. The weaker than modern ENSO signal in Tahiti coral δ 18 O during HS1 ( Fig. 3d,e ) along with the stronger than modern ENSO signal in coral Sr/Ca ( Fig. 3a,b ) implies coherent SST and salinity variations on ENSO timescales during HS1, as the SST variations inferred from Sr/Ca also affect δ 18 O, with positive Tahiti SST anomalies being accompanied by positive salinity anomalies during El Niño events at that time. Our findings suggest that, over the time window represented by the HS1 coral, the effect of the SPCZ and/or the southwestern tropical Pacific salinity front on Tahiti salinity was stronger than today on ENSO timescales, probably indicating a slight displacement and/or intensification of these atmospheric and/or oceanic features. However, we emphasize that we consider the stronger than modern ENSO signal in Tahiti coral Sr/Ca-based SST during HS1 as our most robust finding. As our record is currently unique for interannual tropical Pacific SST variability during HS1, we utilize the only available study of ENSO behaviour during HS1 performed with a comprehensive climate model (CCSM3) [37] . We note that shortcomings of CCSM3 in representing observed modern ENSO variability include a too narrow spatial SST maximum along the equator and a dominant ~2-year period instead of the observed 2–7 year band [37] , [38] . For Tahiti, the simulation indicates an ~20% higher standard deviation of monthly SST anomalies in the interannual ENSO band relative to today ( Fig. 4 ), which is similar to the coral-based estimate. Moreover, the simulation indicates an enhancement of interannual variability of the entire ENSO phenomenon during HS1, and identifies AMOC weakening under glacial boundary conditions as the cause [37] . The AMOC weakening is associated with low SST anomalies in the tropical and subtropical North Atlantic. As a consequence, changes in the east-west SST gradient between the tropical Atlantic and Pacific induce an anomalous Walker circulation and positive trade-wind anomalies across Central and northern South America [39] , [40] . This atmospheric bridge leads to a weakened cross-equatorial SST contrast in the eastern tropical Pacific, accompanied by a weakening of the annual SST cycle in this region and increased interannual ENSO variability [37] , consistent with simulations under modern boundary conditions [40] , [41] , [42] . Whereas the simulation [37] reproduces the increased interannual ENSO variability in Tahiti SST inferred from our HS1 coral, no conclusion can be drawn from the coral with respect to the simulated overall enhancement of ENSO variability during HS1. However, our coral-based results do not necessarily exclude a potential enhancement. Furthermore, the simulation suggests that the Tahiti cooling during HS1, inferred from mean coral Sr/Ca, is not a local feature, but forms part of a Pacific-scale cooling in response to glacial boundary conditions, which is consistent with SST reconstructions from Pacific sediments [22] , [23] , [24] ( Supplementary Fig. S9 ). 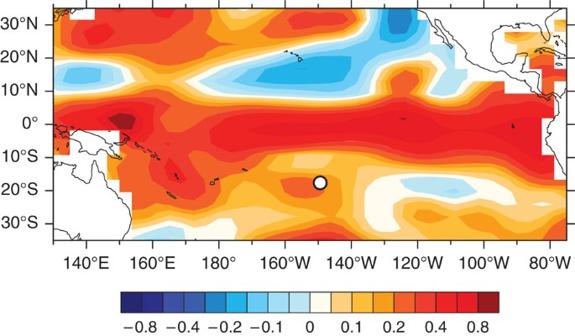Figure 4: Climate model results for Heinrich Stadial 1. Relative response of Pacific interannual SST variability for HS1 simulated by the coupled general circulation model CCSM3 (ref.37). The difference between HS1 and modern climate relative to the latter is shown for the standard deviation (s.d.) of modelled monthly SST anomalies in the interannual El Niño-Southern Oscillation band of CCSM3 (1.5–7 years). A value of 0.2 indicates a 20% higher s.d. of interannual SST anomalies during HS1 relative to modern conditions, for example, near Tahiti (white dot). A ~78% higher s.d. of interannual SST anomalies is indicated for the NINO3.4 region in the central equatorial Pacific (170°–120°W, 5°N–5°S). For the relevant areas in the equatorial Pacific and near Tahiti, the difference between the s.d. for HS1 and modern climate is statistically significant at the 90% level using an F-test (for details seeSupplementary Fig. S12). Note the irregular contour interval. Figure 4: Climate model results for Heinrich Stadial 1. Relative response of Pacific interannual SST variability for HS1 simulated by the coupled general circulation model CCSM3 (ref. 37 ). The difference between HS1 and modern climate relative to the latter is shown for the standard deviation (s.d.) of modelled monthly SST anomalies in the interannual El Niño-Southern Oscillation band of CCSM3 (1.5–7 years). A value of 0.2 indicates a 20% higher s.d. of interannual SST anomalies during HS1 relative to modern conditions, for example, near Tahiti (white dot). A ~78% higher s.d. of interannual SST anomalies is indicated for the NINO3.4 region in the central equatorial Pacific (170°–120°W, 5°N–5°S). For the relevant areas in the equatorial Pacific and near Tahiti, the difference between the s.d. for HS1 and modern climate is statistically significant at the 90% level using an F-test (for details see Supplementary Fig. S12 ). Note the irregular contour interval. Full size image Our fossil coral drilled offshore Tahiti by IODP Expedition 310 indicates that significant interannual SST variability at typical ENSO periods occurred in the tropical South Pacific during HS1, an interval of the last glacial termination that was characterized by extreme cold conditions in the North Atlantic region and a weakening of the AMOC. This is different from today where the ENSO influence on Tahiti SST is weak. Our results suggest a greater ENSO influence in the South Pacific during HS1, related to a southward expansion or shift of ENSO SST anomalies. Our new coral record indicates that ENSO was operating and that interannual ENSO variability was pronounced during HS1. Clearly, more proxy records of interannual tropical Pacific SST variability and model simulations for this critical interval of the last glacial termination are necessary. Our evidence of tropical Pacific SST characteristics in an extreme climate of the past can help to constrain climate models for more reliable projections under future climate change. Diagenetic investigations The preservation of the fossil coral skeleton is comparable to a modern Tahiti Porites ( Supplementary Figs S1 and S2 ). Encrusting microbialites were identified at the outer margin of the fossil coral as high-density areas in X-radiographs. An unaffected area was selected for analysis and investigated using powder X-ray diffraction, petrographic thin sections and SEM. Five conventional X-ray diffraction analyses along the microsampling transect indicate <0.5% calcite (the detection limit). Five petrographic thin sections and SEM analyses indicate excellent preservation of primary porosity, with no evidence for secondary aragonite or calcite cements ( Supplementary Figs S3 and S4 ). Near the core top, SEM suggests slight skeletal dissolution and this section was rejected. In some areas, SEM reveals a slightly rougher skeletal surface compared with modern Tahiti Porites , probably representing very minor dissolution. The skeletal area identified as well preserved was used for microsampling, geochemical analyses and dating. More than two hundred 15–20-μm diameter LA-ICP-MS analyses of polished coral pieces from a representative section of the microsampling transect also indicate no diagenetic cements. Pieces were vacuum impregnated with epoxy resin in a 25-mm diameter round block. Once cured, the block was ground using Al oxide powder to obtain the desired cross section before the surface was finely polished with metallographic grinding paper followed by diamond pastes. Between polishing steps, blocks were briefly ultrasonically cleaned in Milli-Q H 2 O buffered with ammonium hydroxide to pH ~10. Analyses were conducted at the University of Bremen using an Element 2 sector field ICP-MS in low-resolution mode, which was optimized for sensitivity, low oxide production (ThO/U <0.5%), and element fractionation (U/Th 1.0–1.1) by ablation of a NIST 612 glass. LA was performed using a solid state 193 nm laser pulsed at 10 Hz with an irradiance of ~0.6 GW/cm 2 for 30–40 s. The time-resolved signals ( Supplementary Fig. S5 ) of 24 Mg and 88 Sr were background subtracted and internally standardized to 43 Ca to account for variations in ablation yield. Twenty seconds of signal from the period with the most stable Sr/Ca ratio were filtered three times with a 2-σ outlier rejection and averaged for each analysis. Calibration of measured element/Ca ratios was performed using a NIST 610 glass and COCAL calcite powder standard [43] . The precision of the LA-ICP-MS technique was estimated by repeat analysis of a pellet of the JCp-1 coral powder [44] during each analytical session and was generally <10 and <5% (s.d. of mean, 1σ) for Mg/Ca and Sr/Ca respectively. To allow direct comparison of the laser and solution data, laser-derived element/Ca ratios were adjusted by the amount required to match the mean of the laser analyses to that of the solution JCp-1 analyses. These adjustments were typically 0.2 and 0.4 mmol mol −1 for Mg/Ca and Sr/Ca, respectively. LA analyses were conducted across skeletal elements perpendicular to the centres of calcification (COCs). As previously observed in modern corals [45] , COCs are visible as dark patches in polished sections as they are slightly depressed and thus less polished and less reflective. After selecting a section with exposed COCs, a 50-μm spot was scanned across the skeletal element to clean the surface, before a transect of 15–20 μm diameter spots was analysed along the pre-ablated track ( Supplementary Fig. S6 ). A total of 36 transects were analysed along a 38-mm section of the fossil coral and the data are compiled in Supplementary Fig. S7 . In contrast to previous studies of deglacial age fossil corals from Tahiti [14] , [46] , we found no pore fillings to attempt to analyse in our HS1 coral ( Supplementary Fig. S6 ). Instead, we use values from the literature for the composition of secondary aragonite cements and altered COCs [47] , [48] ( Supplementary Fig. S7 ). Mg/Ca ratios are a particularly useful indicator of secondary aragonite and high-Mg calcite cements (for example, ref. 14 ). The >200 measurements clearly demonstrate the absence of secondary aragonite on this length scale. In fact, only one data point approaches the diagenetic aragonite field defined by ion probe studies of a similar length scale to our laser analyses [47] , [48] . The variability of the micron-scale measurements of our fossil coral compares well with that observed by ion probe and nanoSIMS studies of modern Porites corals [45] , [49] , [50] suggesting the original high-resolution biomineralization signal is preserved. Coral dating U-Th analyses were performed using a VG-54 thermo-ionization mass spectrometer equipped with a 30-cm electrostatic analyser and a pulse-counting Daly detector at CEREGE [18] , [51] . Two highly consistent U-Th ages of 15.006±0.065 and 14.992±0.027 kyr BP were determined on two aliquots of the fossil coral, indicating that the coral grew at 14.994±0.025 kyr BP (ages are given relative to AD 1950). Initial ( 234 U/ 238 U) 0 values are highly consistent with a mean value of 1.1453±0.0009 (2σ). This value is within the larger range adopted by the IntCal Group [52] as isotopic screening criterion in the 0–17 kyr interval (( 234 U/ 238 U) 0 = 1.1452±0.0048, 2σ), as a necessary condition for closed system behaviour of U-series isotopes [52] ( Supplementary Table S1 ). Correction for detrital 230 Th is negligible because 232 Th concentrations were <0.5 p.p.b. Powder X-ray diffraction analyses conducted on three distinct slides for each aliquot using a method for detecting and quantifying very low calcite contents [53] indicate ≤0.5% calcite. Two 14 C measurements at the coral's base and centre processed at Laboratoire de Mesure du Carbone 14 (Saclay, France) indicate ages of 15.072±0.130 and 14.964±0.178 cal kyr BP (1σ), in excellent agreement with the U-Th age. Conventional 14 C ages were converted to calibrated ages (cal kyr BP relative to AD 1950) using CALIB6.0 software [54] , the Marine09.14C dataset [55] , a ΔR=−100 (ref. 56 ), and are reported as the midpoint of the 1σ range. All data indicate good preservation of this coral and provide unquestionable chronological constraints on its growth period to be older than the onset of the Bølling warming. Coral records Microsampling of coral skeleton, δ 18 O analyses, chronology construction and monthly interpolation were carried out at the University of Bremen following established methods [27] . Using a 0.7-mm diameter drill bit, an average of 26 samples per year were obtained from the fossil coral by continuous spot-sampling along a single transect. For Sr/Ca analyses a 0.20–0.32-mg split of the sample powder that was used for δ 18 O analyses was dissolved in 7 ml 2% suprapure HNO 3 containing 1 p.p.m. Sc as internal standard. The Ca concentration of dissolved samples was 5–15 p.p.m. Measurements were performed on a Perkin-Elmer Optima 3300R simultaneous radial ICP-OES using a CETAC U5000-AT ultrasonic nebulizer at the University of Bremen. Element wavelengths were detected simultaneously in three replicates (Ca 317.933 nm, Ca 422.673 nm, Sr 421.552 nm, Sc 361.383 nm, Mg 280.271 nm). Ca concentrations measured on an atomic line (422.673 nm) were averaged with the concentrations from an ionic line (317.933 nm) to compensate for possible sensitivity drift in a radial ICP-OES. Calibration standards were diluted from a master standard with a Sr/Ca ratio of 9.099 mmol mol −1 . A control standard set had Ca concentrations of 15 p.p.m. and varying Sr concentrations yielding Sr/Ca ratios of 8.6–10 mmol mol −1 . Measurements of a laboratory coral standard after each sample allowed offline correction for instrumental drift. Relative standard deviation of the Sr/Ca determinations was better than 0.2%. Nine aliquots of the Porites coral powder reference material JCp-1 (ref. 44 ) were treated like samples and the average Sr/Ca value obtained during the course of this study was 8.924±0.014 mmol mol −1 . The approximately fortnightly coral Sr/Ca and δ 18 O records were filtered using a 2-point running mean, a common procedure for coral records with comparable resolution [26] , [57] . For chronology construction, annual Sr/Ca maxima were set to August (on average the coolest month) and annual Sr/Ca minima to March (on average the warmest month). The resulting records were interpolated to a monthly resolution for comparison with instrumental climate data and other coral records. Proxy calibration An average of >17 samples per year was obtained from our modern Porites coral (TAH-95) by continuous spot-sampling. Sr/Ca and δ 18 O analyses were performed at the University of Bremen following the same procedures as for the fossil coral. The seasonal maxima and minima in the Sr/Ca record of the modern coral were tied to the corresponding extreme values in a monthly record of local SST (1986–1991) measured on the ocean side of the barrier reef [31] , ~850 m from the coral site ( Supplementary Fig. S8 ). A linear least-squares regression was then carried out for monthly interpolated Sr/Ca and monthly SST data (SST defined as independent variable), giving a relationship of: The same procedure was applied to the coral δ 18 O record, giving a relationship of: Climate model simulations The simulations with the Community Climate System Model (CCSM3), an ocean-atmosphere-sea ice-land surface general circulation model, are described in ref. 37 . A present-day control simulation using the standard CCSM3 model set-up [38] was performed. All simulations were carried out at Norddeutscher Verbund für Hoch- und Höchstleistungsrechnen (HLRN, Hannover, Germany). How to cite this article: Felis T. et al . Pronounced interannual variability in tropical South Pacific temperatures during Heinrich Stadial 1. Nat. Commun. 3:965 doi: 10.1038/ncomms1973 (2012).